Genome sequencing of chimpanzee malaria parasites reveals possible pathways of adaptation to human hosts Plasmodium falciparum causes most human malaria deaths, having prehistorically evolved from parasites of African Great Apes. Here we explore the genomic basis of P. falciparum adaptation to human hosts by fully sequencing the genome of the closely related chimpanzee parasite species P. reichenowi , and obtaining partial sequence data from a more distantly related chimpanzee parasite ( P. gaboni ). The close relationship between P. reichenowi and P. falciparum is emphasized by almost complete conservation of genomic synteny, but against this strikingly conserved background we observe major differences at loci involved in erythrocyte invasion. The organization of most virulence-associated multigene families, including the hypervariable var genes, is broadly conserved, but P. falciparum has a smaller subset of rif and stevor genes whose products are expressed on the infected erythrocyte surface. Genome-wide analysis identifies other loci under recent positive selection, but a limited number of changes at the host–parasite interface may have mediated host switching. P lasmodium falciparum causes the overwhelming majority of human malaria mortality, and is only distantly related to the other major human Plasmodium species. Until recently, the only known close relative of P. falciparum was P. reichenowi, a malaria parasite of chimpanzees that is morphologically so similar to P. falciparum that they were initially thought to be the same species [1] . In recent years, this simple view of the origins of P. falciparum has been comprehensively overhauled by a series of molecular studies that have revealed an unexpected diversity of P. falciparum related parasites in African apes [2] , [3] , [4] , [5] , [6] . These studies establish that all human P. falciparum parasites fall as a single cluster within a broader network of ape parasites, now collectively referred to as the Laverania subgenus, and the closest relative and likely origin of human P. falciparum is a clade of parasites found in western gorillas [3] . Laverania parasites appear to be largely host specific, with individual clades infecting only chimpanzees or gorillas, even when the apes are sympatric, and there are at least three clades infecting both chimpanzees ( P. reichenowi, P. gaboni and P. billcollinsi ) and gorillas ( P. praefalciparum, P. adleri and P. blacklocki ). However, to date, comparisons between these new Laverania clades have relied primarily on mitochondrial genome sequences, with only fragments of the nuclear genome amplified and sequenced. An understanding of the forces driving the radiation of the Laverania subgenus, and the extent of genomic diversity between Laverania clades, awaits the generation of whole-genome sequences for all species. While low-coverage capillary sequence data has been generated for P. reichenowi previously [7] , no complete genome has been generated for any Laverania parasite other than P. falciparum In this study, we present the first comparative genomic analysis of Laverania parasites by comparing high-quality genome sequences of P. reichenowi P. falciparum [8] and partial genome sequence data from P. gaboni , another species of the Laverania subgenus, obtained from a chimpanzee blood sample following a routine health check. Our analyses show that these genomes are essentially co-linear in the core central regions, allowing us to focus on the small number of significant differences. The most striking of these involve genes associated with red cell invasion implicating them in determining host specificity. In the highly polymorphic multigene families located in the subtelomeric regions, we observe one-to-one orthology in some ( PHIST and FIKK ), a commonality in the basic architecture of the var family that is involved in antigenic variation and significant copy number variation in the rif and stevor families [4] . A high-quality reference genome for P. reichenowi was produced from Illumina reads using de novo assembly and post hoc improvement ( Supplementary Methods and Supplementary Fig. 1 ). The 24 Mb sequence extends into the subtelomeres on four chromosomes ( Supplementary Fig. 2 ) and encodes 5,731 genes ( Fig. 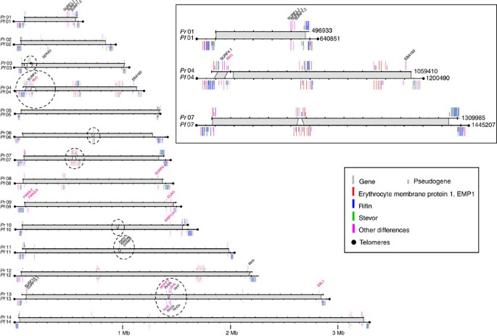Figure 1: Alignment of theP. reichenowiCDC andP. falciparum3D7 genomes. The 14 chromosomes of the nuclear genome are aligned and regions with shared synteny are shown shaded in grey, divergent loci are circled. Variable extracellular multiprotein families, Stevors (green), Rifins (blue) and erythrocyte membrane protein 1 (red), are shown and pseudogenes for each of these multigene families are shown (shorter lines). Differentially distributed genes or pseudogenes (Supplementary Data 1) are shown in pink with annotations highlighting thePrCDC difference and pseudogenes highlighted with pink text. The values on the right side of the chromosomes indicate the total length of the assembled sequence scaffold in base pairs. 1 and Table 1 ). Excluding the subtelomeres, the genome is almost completely co-linear with P. falciparum and share almost identical gene content emphasizing their recent shared ancestry ( Fig. 1 ). The vast majority of these ~5,000 ‘core’ genes are common to both parasites, with only three genes present in P. reichenowi that are missing in P. falciparum and only one in P. falciparum that is absent from P. reichenowi ( Supplementary Fig. 3 ). In addition, 19 intact genes in the chimpanzee parasite are pseudogenes in P. falciparum and there are 16 genes for which the reverse is the case ( Supplementary Data 1 and Supplementary Fig. 4 ). Twenty-seven orthologous loci contain pseudogenes in both species, and these vary in their degree of coding sequence degeneracy. Figure 1: Alignment of the P. reichenowi CDC and P. falciparum 3D7 genomes. The 14 chromosomes of the nuclear genome are aligned and regions with shared synteny are shown shaded in grey, divergent loci are circled. Variable extracellular multiprotein families, Stevors (green), Rifins (blue) and erythrocyte membrane protein 1 (red), are shown and pseudogenes for each of these multigene families are shown (shorter lines). Differentially distributed genes or pseudogenes ( Supplementary Data 1 ) are shown in pink with annotations highlighting the Pr CDC difference and pseudogenes highlighted with pink text. The values on the right side of the chromosomes indicate the total length of the assembled sequence scaffold in base pairs. Full size image Table 1 Comparison of genome statistics between P. reichenowi CDC and P. falciparum 3D7. Full size table Significant differences were anticipated for genes that function at the host–parasite interface. In P. falciparum, many of these genes are subtelomeric, most notably in a number of multigene families that encode proteins that are exported into the host erythrocyte. Plasmodium subtelomeres are highly repetitive and difficult to assemble, but we were able to assemble the majority of P. reichenowi coding sequences in these regions, and thereby produced the first complete genome sequence for a Laverania parasite other than P. falciparum . In several multigene families of exported proteins, including the PHIST and FIKK families [9] , clear orthologues could be identified for almost all genes between P. falciparum and P. reichenowi ( Fig. 2a ). The few exceptions ( Fig. 2a ) occurred where P. reichenowi orthologues were pseudogenes ( Supplementary Fig. 5 ). 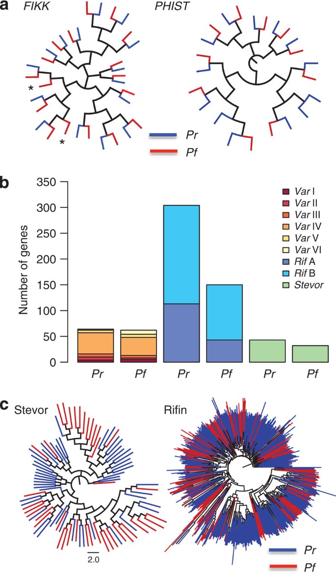Figure 2: Number and organization of multigene families encoding proteins exported into the infected erythrocyte. (a) Dendrograms of the exported kinase (FIKK) and PHIST domain containing proteins showing one-to-one orthologous pairing betweenP. reichenowi(blue) andP. falciparum(red). TwoP. falciparum FIKKgenes have no protein coding orthologue (starred) because the homologous genes have become pseudogenes inP. reichenowi(Supplementary Fig. 5). (b) Distribution of the number of intact members of thevar,rifandstevorfamilies within each defined subclass in bothP. falciparum(Pf) andP. reichenowi(Pr). (c) Dendrograms of therifandstevorprotein families inP. falciparumandP. reichenowi, showingP. reichenowi-specific expansions in both cases. Figure 2: Number and organization of multigene families encoding proteins exported into the infected erythrocyte. ( a ) Dendrograms of the exported kinase (FIKK) and PHIST domain containing proteins showing one-to-one orthologous pairing between P. reichenowi (blue) and P. falciparum (red). Two P. falciparum FIKK genes have no protein coding orthologue (starred) because the homologous genes have become pseudogenes in P. reichenowi ( Supplementary Fig. 5 ). ( b ) Distribution of the number of intact members of the var , rif and stevor families within each defined subclass in both P. falciparum ( Pf ) and P. reichenowi ( Pr ). ( c ) Dendrograms of the rif and stevor protein families in P. falciparum and P. reichenowi , showing P. reichenowi -specific expansions in both cases. Full size image The extremely polymorphic var multigene family encodes the PfEMP1 proteins that are central to the pathogenesis and persistence of malaria infection in humans where their expression on the surface of infected erythrocytes mediates adherence to a variety of receptors on different host cell types [10] , [11] , [12] . Surprisingly, between P. falciparum and P. reichenowi, var genes are conserved both in number ( Table 2 ) and broadly, in terms of their organization and size ( Fig. 2b ). PfEMP1 proteins are highly polymorphic and are composed of varying numbers and classes of Duffy-binding-like (DBL) domains and cysteine-rich interdomain regions (CIDR), that mediate adhesion, with the amino terminal DBL domain (DBLα) being the most conserved [13] . The relative orders of these domains vary markedly between gene copies in P. falciparum, but the most frequent arrangement in P. falciparum (DBLa-CIDRa-DBLd-CIDRb) was also the second-most abundant in P. reichenowi ( Supplementary Data 2 ). While their overall organization is conserved, individual PfEMP1 sequences were highly divergent between P. reichenowi and P. falciparum , just as they are between P. falciparum strains. However, even here crucial aspects were conserved. The most highly conserved amino acid sequence motif in the P. falciparum DBLα domain, LARSFADIGDI, was completely conserved in P. reichenowi, but based on the limited data available only a variant of this sequence is recognizable in P. gaboni , and the surrounding sequences appear to be more polymorphic ( Supplementary Fig. 6 ). Although the extent of var gene diversity makes direct pairwise comparisons impossible for most of their sequences, P. falciparum DBLα domains can be categorized on the basis of cysteine content, length and semi-conserved motifs into six different classes [13] . All six DBLα classes were evident in P. reichenowi in approximately the same ratios as in P. falciparum ( Fig. 2b and Table 2 ). Table 2 Comparison of gene families between P. reichenowi CDC and P. falciparum 3D7. Full size table In summary, despite the fact that radical polymorphism in var genes is essential for their role in immune evasion, their number, organization and some elements of sequence appear to be conserved between chimpanzee and human parasites. By contrast, we found that the size of the rif and stevor multigene families, which also encode proteins expressed on the surface of infected red blood cells and other stages directly exposed to the host [14] , [15] , is markedly different between the two species. While the function of these genes is not known, homologues are found in all Plasmodium species, implying a universal and ancient role in the relationship between Plasmodium parasites and their vertebrate hosts. There are 568 rif genes in P. reichenowi and only 185 in P. falciparum , with the number of pseudogenes differing by a similar ratio (49 and 27, respectively; Table 2 and Fig. 2b ). The number of stevor genes is also higher in P. reichenowi (66) than in P. falciparum (42). Successful colonization of humans is therefore clearly possible with a much reduced repertoire of these two important multigene families. The relative size of the rif and stevor gene families were the most striking differences between P. reichenowi and P. falciparum at the genome structure level, but having almost complete sequence data for the P. reichenowi genome also enabled us to take a systematic approach to identifying genes that were significantly different in sequence between these two species ( Supplementary Note 1 ), and therefore might be involved in adaptation to human hosts. Unfortunately, a limited representation within the sequencing libraries precluded performing similar systematic analyses in parallel using the P. gaboni genome data ( Supplementary Note 1 and Supplementary Data 3 ). The Hudson–Kreitman–Aguade ratio (HKAr) [16] summarizes the ratio of interspecific nucleotide divergence ( K ) to intraspecific polymorphism ( π ). We used an assembly-based approach and five different P. falciparum strains to enable π and K to be derived for most of the coding sequences in the P. falciparum genome ( n =4,933; Supplementary Data 4 ). The distribution of K values was highly skewed across genes ( Supplementary Fig. 7a ), with a mean of 0.024, whereas for intergenic regions, K values were much higher but less skewed, with a mean of 0.033 ( Supplementary Data 5 ; P =2.2e−16). To identify genes with unusually high levels of polymorphism in P. falciparum and to minimize random sampling variance in the HKAr test, we focussed on loci for which the denominator K had ≥5 fixed nucleotide differences. Coding regions generally contained a lower ratio of polymorphisms to fixed differences than intergenic regions, reflected in lower π / K ratios (coding, mean=0.025, n =4445; intergenic, mean=0.044; Mann–Whitney test, 10 −16 ). Particularly, high HKAr values of over 0.15—likely to reflect diversifying selection within P. falciparum —were seen for 72 coding sequences ( Fig. 3 and Supplementary Data 6 ). Of these, 45 had functional annotations, and 10 of these are considered likely to be associated with erythrocyte invasion [17] , including three members of the merozoite surface protein 3 ( msp3 ) gene family on chromosome 10, a highly variable locus amongst P. falciparum strains ( Supplementary Fig. 8 ). 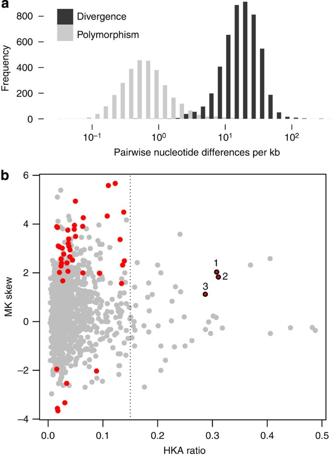Figure 3: Genome-wide scan for genes under selection pressure. WherePf3D7–PrCDC orthologues could be identified, polymorphism was calculated from the alignment of five laboratory clones and divergence was calculated from the pairwise alignment ofPf3D7–PrCDC, respectively (a). From the data ina, McDonald–Kreitman (MK) and Hudson–Kreitman–Aguade ratio (HKAr) values were calculated for every orthologous pair of genes across the two genomes (b). The MK skew is the log (base 2) of the odds ratio of the 2 × 2 contingency table of numbers of non-synonymous versus synonymous polymorphisms among fiveP. falciparumlines divided by numbers of non-synonymous versus synonymous fixed differences betweenP. reichenowiandP. falciparum. Genes with significant MK skew determined by Fisher’s exact test are highlighted in red. The HKAr of nucleotide polymorphism (withinP. falciparum) divided by divergence (betweenP. falciparumandP. reichenowi) is independently distributed from the MK ratio. Individual values for each gene are listed inSupplementary Data 4–7. A threshold of HKAr values >0.15 (dotted line) was used to identify highlight genes under particularly high diversifying selection. Genes with high HKAr, plus significant and high MK skew: (1) apical membrane antigen 1 (PF3D7_1133400); (2) putative conserved membrane protein of unknown function (PF3D7_0104100); and (3) putative conserved membrane protein of unknown function (PF3D7_0710200). Figure 3: Genome-wide scan for genes under selection pressure. Where Pf 3D7– Pr CDC orthologues could be identified, polymorphism was calculated from the alignment of five laboratory clones and divergence was calculated from the pairwise alignment of Pf 3D7– Pr CDC, respectively ( a ). From the data in a , McDonald–Kreitman (MK) and Hudson–Kreitman–Aguade ratio (HKAr) values were calculated for every orthologous pair of genes across the two genomes ( b ). The MK skew is the log (base 2) of the odds ratio of the 2 × 2 contingency table of numbers of non-synonymous versus synonymous polymorphisms among five P. falciparum lines divided by numbers of non-synonymous versus synonymous fixed differences between P. reichenowi and P. falciparum . Genes with significant MK skew determined by Fisher’s exact test are highlighted in red. The HKAr of nucleotide polymorphism (within P. falciparum ) divided by divergence (between P. falciparum and P. reichenowi ) is independently distributed from the MK ratio. Individual values for each gene are listed in Supplementary Data 4–7 . A threshold of HKAr values >0.15 (dotted line) was used to identify highlight genes under particularly high diversifying selection. Genes with high HKAr, plus significant and high MK skew: (1) apical membrane antigen 1 (PF3D7_1133400); (2) putative conserved membrane protein of unknown function (PF3D7_0104100); and (3) putative conserved membrane protein of unknown function (PF3D7_0710200). Full size image As a separate test for non-neutral evolution, we compared polymorphism versus divergence using ratios of synonymous and non-synonymous differences in coding sequences with the McDonald–Kreitman (MK) test [18] . The individual genes with significantly high ratios ( Fig. 3 ; and Supplementary Data 4 and 7 ) may either be under balancing selection (maintaining intraspecific polymorphisms) or under weak negative selection (allowing some nearly neutral polymorphism to be retained but preventing fixed differences). Three genes showed extreme values in both the HKAr and MK test, and encode apical membrane antigen-1—a known polymorphic protein crucial to merozoite invasion—as well as two previously uncharacterized proteins ( Fig. 3b ). An indication of proteins that may have been under positive selection can also be obtained by examining K a/ K s ratios of fixed differences between species. Of the 100 proteins with the highest K a/ K s ratios, 77 have no known function but significantly ( P <0.0001, χ 2 -test for enrichment compared with the genome as a whole) 31 of the 100 have predicted motifs for export into the infected erythrocyte. Six of these proteins are involved in erythrocyte invasion, again emphasizing that the strongest selection pressures is acting on the parasite–erythrocyte interface ( Supplementary Data 4 and 8 ). Introgression between species potentially confounds interpreting evolutionary signatures of selection. However, the lack of evidence that the high HKAr loci are spatially clustered in the genome ( Supplementary Fig. 9 ) and the smooth distribution of K values ( Supplementary Fig. 7b ) suggest that major genetic introgression is not a factor. Genome-wide tests thus identified particular selection pressure on erythrocyte invasion. Moreover, of only 16 genes that are missing or pseudogenes in the P. reichenowi genome, three are members of invasion-associated multigene families, SERA3 , MSP3.8 ( Supplementary Fig. 8 ) and MSRP3 (on chromosomes 2, 10 and 13, respectively; Supplementary Data 1 ) [19] . Both genome-wide tests for selection, as well as gene loss and gain, therefore identify erythrocyte invasion loci as being significantly different between the P. falciparum and P. reichenowi genomes. Erythrocyte recognition is dependent on two multigene families, the reticulocyte-binding-like (RBL) and erythrocyte-binding-like (EBL) proteins. Members of these families have been found in every Plasmodium species sequenced to date and here the differences between P. falciparum and P. reichenowi were particularly striking. Within the five-member EBL family, eba-165 , is a pseudogene in P. falciparum ( Supplementary Fig. 10a ) but not in P. reichenowi [20] , while EBL1 has a substantial deletion in P. reichenowi that may render it non-functional ( Supplementary Fig. 10b ). Similarly, of six RBLs in the P. falciparum genome only three ( Rh2b, Rh4 and Rh5 ) have clear orthologues in P. reichenowi . This analysis confirmed previous observations that Rh1 (ref. 21 ) is a highly divergent pseudogene in P. reichenowi [22] , whereas Rh3 is a pseudogene in P. falciparum [23] but has a complete open reading frame in P. reichenowi [22] . The Rh2 locus on chromosome 13 ( Fig. 4a ) is the most substantially different between the species. P. falciparum , it contains two almost identical genes, PfRh2a and PfRh2b , and a highly degenerate pseudogene, PfRh6 (refs 24 , 25 , 26 ), whereas in P. reichenowi , Rh2b is inverted and there is an inversion and complete divergence of Rh2a with a gene so distinct that we refer to it as PrRh7 . The overall arrangement of the P. reichenowi genomic region is also significantly different, with PrRh2b and PrRh7 lying head to tail and separated by Rh6 , a pseudogene that in P. falciparum lies downstream of Rh2b . Despite the nature of our P. gaboni sample precluding a full-genome assembly, we could identify an orthologue of PrRh2b and PfRh2a ( Fig. 4a ), as well as a close orthologue of PrRh7 , supporting the inference that the inversion/duplication event at this locus has happened only in the P. falciparum branch ( Fig. 4b ). Surprisingly, we found strong evidence that the orthologue of the Pr - and PfRh6 pseudogenes is in fact an intact gene in P. gaboni , suggesting further that changes at this locus had also taken place between the chimpanzee Plasmodium species ( Fig. 4 ). The radical changes in gene identity and organization at this individual invasion gene locus reinforce the whole-genome analysis, and suggest that extensive changes in the erythrocyte invasion repertoire may have accompanied the expansion of Laverania species and their transitions between hosts. 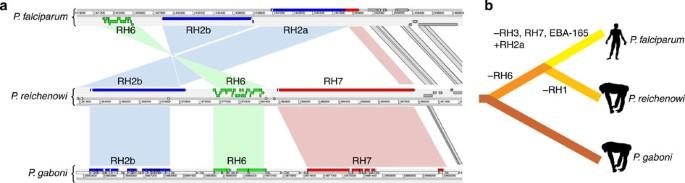Figure 4: Evolution of erythrocyte invasion ligands acrossLaveraniaparasite species. (a) Comparison of the RH locus on chromosome 13 betweenP. falciparum3D7,P. reichenowiCDC andP. gaboni. The forward and reverse DNA strands are shown as thick horizontal lines (grey), with sequence gaps (white boxes), where appropriate. Annotated genes (red/green/blue) are shown above or below the DNA lines, in forward or reverse reading frames, respectively, and connected by coloured quadrilaterals to indicate conservation between homologous genes. At this one locus, there have been two incidents of gene loss (RH7betweenPf3D7 andPrCDC;Rh6between Pg and Pr) and one incident of gene gain (Rh2ainPf). Multiple frameshifts inPrandPfare shown but none could be detected inPg. (b) Stylized phylogram showing the relationship betweenP. falciparum, P. reichenowiandP. gaboni, indicating the incidents of gene loss and gain within theEBLandRhgene families across the species radiation. Figure 4: Evolution of erythrocyte invasion ligands across Laverania parasite species. ( a ) Comparison of the RH locus on chromosome 13 between P. falciparum 3D7, P. reichenowi CDC and P. gaboni . The forward and reverse DNA strands are shown as thick horizontal lines (grey), with sequence gaps (white boxes), where appropriate. Annotated genes (red/green/blue) are shown above or below the DNA lines, in forward or reverse reading frames, respectively, and connected by coloured quadrilaterals to indicate conservation between homologous genes. At this one locus, there have been two incidents of gene loss ( RH7 between Pf 3D7 and Pr CDC; Rh6 between Pg and Pr) and one incident of gene gain ( Rh2a in Pf ). Multiple frameshifts in Pr and Pf are shown but none could be detected in Pg . ( b ) Stylized phylogram showing the relationship between P. falciparum, P. reichenowi and P. gaboni , indicating the incidents of gene loss and gain within the EBL and Rh gene families across the species radiation. Full size image By generating the first complete genome sequence of any non-human Laverania parasite, as well as partial sequence from a second, we have been able to take the first systematic view of differences between these important pathogens, from which the most significant human malaria parasite evolved. Despite the fact that these are distinct species with no evidence of recent introgression, our data show that the genomes of human and chimpanzee Laverania species are remarkably similar. Excluding the subtelomeres, which contain genes associated with antigenic variation and are also highly polymorphic between different P. falciparum genotypes, the genomes are effectively co-linear. Against this strongly conserved ‘background’, differentially distributed genes or diverged genes presented a stark contrast, and we observed two different classes of divergence—genes within the core genome that show strong evidence of selection and differences in multigene families in the subtelomeric regions. In the case of multigene families, many families such as the PHIST and FIKK genes show clear orthology between P. reichenowi and P. falciparum . Rodent Plasmodium genomes contain only a single FIKK gene, so it appears that both these families expanded before the P. reichenowi/P. falciparum divergence, and selection pressure to preserve the expanded number of genes has been maintained after speciation. Surprisingly, similarities between P. falciparum and P. reichenowi multigene families extended to the highly polymorphic var gene family that is central to parasite survival in the vertebrate host through mediating the process of antigenic variation and immune evasion. Although sequence similarity is low between the two species (as it is between different P. falciparum isolates), the relative ratio of different DBLα sequence types in P. reichenowi is very close to that in the human parasite, suggesting that maintaining the relative ratios of DBLα classes is functionally important in infections of both apes and humans. A previous analysis [27] of low coverage genome survey sequencing data from P. reichenowi [7] showed that many of the basic building blocks are conserved in DBLα, but this complete genome sequence shows for the first time conservation in the domain type ratios and their organization. Our limited data from P. gaboni provide the first indication that there might be more sequence variation within the var gene family in this organism, although traces of the same conserved short amino acid block clearly remain. The most notable difference in the gene complement in the subtelomeres is seen between the rif and stevor multigene families where the numbers are much lower in the human parasite. The rif genes have previously been divided into A and B subtypes based on the presence or absence of a 25-codon insert in the second exon [28] . Despite the difference in numbers of rif genes, both species contain A and B subtypes with ratios of A and B of 0.6 and 0.4 in P. reichenowi and P. falciparum, respectively, supporting a gene family split that predates speciation ( Fig. 2b ). Orthologues of the rif and stevor families are present in all Plasmodium spp. sequenced to date and are known collectively as the Plasmodium interspersed repeat ( pir ) family. It is noteworthy that P. falciparum has one of the lowest complements of the pir family of any species yet sequenced. We believe that this is a genuine difference between species rather than a chance finding due to copy number variation in P. falciparum . Although only a single clone of P. falciparum is fully sequenced and assembled, draft assemblies are available for a number of other strains (IT, HB3 and Dd2). Despite the fact that the subtelomeres are incompletely assembled in these sequences, searching the assembled contigs for motifs specific to each of these rif and stevor multigene families results in very similar numbers for all P. falciparum strains. A recent contraction of the rif and stevor families in the human parasite ( Fig. 2c ) is therefore likely and, unlike other exported multigene families, these two families appear to be under quite different pressures in P. falciparum and P. reichenowi . Evolution has thus had different effects on subtelomeric multigene families, but critically the founder members and basic organization occurred before the emergence of P. falciparum . With respect to genes in the core region of the genome, we found it striking that among the 100 most divergent genes between species, the majority (77) encode proteins of unknown function. Only 38% of genes in the P. falciparum genome have this definition, highlighting that the least explored content of the genome includes genes that may have important roles relating to host differences. This work therefore immediately identifies a number of new genes for which functional work is urgently required. Of the genes with ascribed functions, six are known to be involved in erythrocyte invasion, and tests for genes under selection (MK and HKAr) also identified several genes associated with this essential step in the Plasmodium life cycle. These widespread changes in invasion loci is most notable at the Rh2 locus on chromosome 13 where significant rearrangement and diversification has occurred, not only just between P. falciparum and P. reichenowi but also between the two chimpanzee parasite species, P. reichenowi and P. gaboni . Given the otherwise relatively limited changes both in the core genome and in the functional subdivisions within the exported protein families, we hypothesize that changes in the sequence and arrangement of genes in the EBL and RBL family may be directly associated with Laverania host adaptation. Support for this hypothesis with respect to the Rh genes comes from the recent data that shows that Rh5 , a member of the RBL family that is essential for erythrocyte invasion in P. falciparum and has previously been implicated in host specificity [29] , [30] , is strikingly primate specific in its receptor-binding preferences [31] . Further studies will be needed to directly establish the role that these new RBL family members also have a role in primate-specific erythrocyte recognition, and thus may contribute to Laverania host restriction. The recent discovery of multiple species of P. falciparum related parasites in African apes has raised numerous questions about the potential of these Laverania parasites to act as zoonotic pathogens of humans. While molecular surveys and epidemiological work will contribute to the answers to these questions [32] , a molecular understanding of the factors that restrict Laverania parasites to specific hosts is also needed. This first complete genome analysis of a Laverania parasite very clearly identifies changes at the host–parasite interface during the blood stages of their life cycle, both during erythrocyte invasion and on the surface of the infected erythrocyte, as well as a short list of genes of unknown function, as potential key contributors to host specificity. The relative contribution of each of these candidates to speciation and host switching awaits further functional study. P. reichenowi genome sequencing The only extant isolate of P. reichenowi ( Pr CDC) was obtained from a chimpanzee imported to the United States of America from the Belgian Congo (now the Democratic Republic of Congo) in the 1950s (ref. 33 ). Before commencement of the present study, parasites were collected (in 2001), with approval of the Institutional Ethics Committee and according to Dutch law, from a chimpanzee called Dennis that had been infected with P. reichenowi from a chimpanzee called Oscar at the Center for Disease Control, Atlanta. Twelve days after infection, parasitemia had reached 0.5%, and blood was collected and filtered to reduce white blood cell numbers (Plasmodipur, the Netherlands). The chimpanzee was subsequently cured of infection by treatment with chloroquine. DNA was isolated from infected erythrocytes using the PureGene gDNA isolation kit (Gentra Systems, Minneapolis, USA) and subsequently stored at 4°C. Genomic DNA was sheared into 300–500 base pair (bp) fragments by focused ultrasonication (Covaris Inc., Woburn, USA). Amplification-free Illumina libraries were prepared [34] and 76-bp-end reads were produced on an Illumina Genome Analyzer IIx following the manufacturer’s standard cluster generation and sequencing protocols [35] . A 3–4-kb mate-pair library was prepared using the Illumina mate-pair library prep kit (v1) and sequenced as above. In total, 202 million reads were produced and deposited in the European Nucleotide Archive with the accession number ERP000299 . P. gaboni genome sequencing During a routine medical investigation, P. gaboni was isolated from a young male chimpanzee in Koulamoutou, Ogooué-Lolo Province, Gabon, and conserved in 7 ml EDTA vacutainers. The investigation was approved by the Government of the Republic of Gabon and by the Animal Life Administration of Libreville, Gabon (no. CITES 00956). All animal work was conducted according to relevant national and international guidelines. Red cells and plasma were separated by centrifugation and stored at −20°C until transportation to the Centre International de Recherches Médicales de Franceville, Gabon, where they were stored at −80 °C until processed. To overcome host contamination, flow cytometry and cell sorting [36] were performed. Two sets of 10,000 parasite nuclei (Gab.1.4. and Gab.1.5.) were obtained. Whole-genome amplification was performed on each set using an Illustra GenomiPhi V2 DNA Amplification Kit (GE Healthcare, Uppsala, Sweden), followed by purification through Illustra Sephadex G-50 DNA Grade F columns (GE Healthcare). The two final products were then pooled for subsequent sequencing. Genomic DNA was sheared into 300–400-bp fragments by focused ultrasonication (Covaris Adaptive Focused Acoustics technology (AFA Inc., Woburn, USA)). A standard Illumina library was then prepared following the manufacturer’s protocol [35] . Using an Illumina Genome Analyzer IIx, 76-bp-end reads were initially produced from the library. The depth of coverage was subsequently increased using an Illumina HiSeq 2000 to produce 76-bp-end reads. In total, 447 million raw reads were produced and deposited in the European Nucleotide Archive with the accession number ERP000135 . Limited template coverage of the P. gaboni genome precluded a systematic genome-wide analysis of sequence variation, but the limited number of genes for which we could calculate K a/ K s ratios are given in Supplementary Data 3 . Assembly of P. reichenowi Before sequence assembly, contaminating host-derived sequences were excluded by mapping to the chimpanzee genome using SSAHA [37] and BWA [38] . Putative sequencing errors in the reads were removed using SGA [39] . A working reference of P. reichenowi was produced by iteratively mapping the Illumina reads against the P. falciparum 3D7 genome ( Pf 3D7) and changing the sequence of the latter to match apparent fixed differences using iCORN [40] . Against this working reference, P. reichenowi reads were remapped using SMALT and a guided assembly was performed using Velvet Columbus [41] . Contigs were joined into scaffolds using SSPACE [42] and paired reads from the PCR-free the amplified 3 kb libraries. Scaffolds ≥500 bp were ordered and oriented against the Pf 3D7 reference genome using ABACAS [43] and gaps closed by further mapping of Illumina reads using IMAGE [44] . Where contig–contig joins were supported by <3 mapped mate pairs, scaffolds were broken. Iteratively remapping Illumina reads and correcting erroneous bases using iCORN further improved the P. reichenowi assembly. Assembly of P. gaboni The assembly of P. gaboni resulted in many fragmented small contigs owing to the low amount of template DNA and high level of host and adapter contamination. Although we tested the same methodology as used with the Pr CDC genome (that is, transforming the genome), better results were obtained by assembling the corrected reads de novo using Velvet. The P. gaboni assembly is available from: ftp://ftp.sanger.ac.uk/pub/pathogens/Plasmodium/gaboni/Assembly/Version1/. Assembly of P. falciparum laboratory clones The genome of P. falciparum IT clone was produced by Illumina sequencing from a PCR-free small fragment library together with a 2.5-kb mate-pair library. The data were assembled de novo , improved using the PAGIT pipeline [45] and stored in GeneDB. For the three other laboratory clones (DD2, HB3 and 7G8), read quality was insufficient to produce complete de novo assemblies, as many coding regions were not generated. Therefore, a morphing approach was used, whereby reads from the above genomes were iteratively mapped to the genome of 3D7 and SNPs, and small indels incorporated until no further differences could be called [40] . Raw reads of the four isolates are ERS013737 (IT), ERS005005 (DD2), ERS010000 (HB3) and ERS006631 (7G8). The annotated assemblies for the four laboratory clones can be found at the following FTP sites: ftp://ftp.sanger.ac.uk/pub/pathogens/Plasmodium/falciparum/IT_strain/version_2/June_2012/ , ftp://ftp.sanger.ac.uk/pub/pathogens/Plasmodium/falciparum/DD2/Assembly/V1_morphed , ftp://ftp.sanger.ac.uk/pub/pathogens/Plasmodium/falciparum/7G8/Assembly/V1_morphed , ftp://ftp.sanger.ac.uk/pub/pathogens/Plasmodium/falciparum/HB3/Assembly/V1_morphed. Annotation From 5,418 genes in Pf 3D7, 5,111 were transferred to P. reichenowi using RATT [46] . In regions with no shared synteny, genes were predicted ab initio using Augustus [47] , with the transferred gene models as a training set, and manually inspected in Artemis. P. gaboni was not annotated owing to its highly fragmented state and was instead used for focused comparisons where contigs were aligned to specific loci of interest. To annotate the laboratory clones, annotation was transferred using RATT and, in the case of P. falciparum IT, gene models were systematically corrected manually using Artemis and the Artemis Comparison Tool [48] . The alignments for genes with extreme HKAr or MK values (below) were manually checked, and in some cases resulted in additional edits to gene models to update their structures in accordance with the June 2012 annotation. Putative exported proteins were predicted using Exportpred v 2.0 (ref. 49 ). Analysis of gene family trees For each gene family ( Surfin, PHIST, FIKK, rif and stevor ), we constructed phylogenetic trees. Multiple alignments of each family were produced with Clustal W [50] . For the Rifin and Stevor families, only full-length uninterrupted translations were used. Four P. reichenowi Rifins were excluded from analysis owing to internal gaps within their sequences, and in both P. reichenowi (PRCDC_1038200 and PRCDC_0004700) and P. falciparum (PF3D7_0401600) contain divergent Rifin sequences that align poorly to either type A or type B Rifins. For other families, protein sequences that differed in length by >15% from the median were excluded, along with pseudogenes. From the obtained alignment, trees were calculated with PhyML version 3.0.1 (ref. 51 ) (LG model, aLRT branch support; optimized ‘Across site rate variation’ NNI Tree searching operation; BioNJ Starting tree (enabling optimized tree topology)). For colouring, we used a PERL script and FigTree ( http://tree.bio.ed.ac.uk/software/figtree/ ). Analysis of var genes The var genes in P. reichenowi were annotated during the automatic functional annotation. In general, the var genes of Pr CDC are longer than those of Pf 3D7 but not significantly different to P. falciparum when other isolates are taken into account. Not all of them are completely assembled as many are missing the second, highly conserved, exon ( Supplementary Data 2 ). Two var genes that are known to be more conserved in P. falciparum isolates than the rest of the repertoire— var1csa and var2csa (the latter known to be associated with malaria in pregnancy [52] )—were also present but differed in length. Compared with its Pf 3D7 orthologue, the var2csa gene of Pr CDC is ~5 kb shorter and runs into telomeric repeats despite being located in an interstitial region. Pr VAR1CSA is 1,584 bp longer than its Pf 3D7 orthologous. The similarity between Pf 3D7 and Pr CDC also includes the arrangement of the internal var gene clusters on chromosomes 4, 7, 8 and 12. The internal var gene locus on Chr 6 in 3D7 ( var gene PF3D7_0617400) is, however, not present in Pr CDC. On chromosome 3, the var gene locus that is a pseudogene in 3D7 (PF3D7_0302300) is intact in Pr CDC. The var -encoded protein domains were classified using the VARdom server [53] and the output parsed with a bespoke PERL script. DBLα domains were classified according to ref. 54 , using a bespoke PERL script ( Supplementary Data 2 ). To identify var genes in P. gaboni , we also searched the P. gaboni assembly for matches to the P. falciparum var genes using BLASTX (E-value cutoff of 10 −6 ). All contigs that hit a 3D7 var gene were extracted and open frames ≥1,500 bp were identified. This resulted in 15 var gene fragments, with a mean length of 973 amino acids (largest 3130 amino acids). The largest var gene had as first hit a weak similarity to the var1csa of P. falciparum IT and 3D7. The putative var genes of P. gaboni were aligned with those of Pr CDC and Pf 3D7 using Clustal W. Interestingly, the conserved LARSFADIGDI motif from the latter two species, which is present in the first DBL domain and has been universally used for the design of PCR primers, appears to be different and degenerate in P. gaboni (A[LIM][KR][YN]SF[A/Y]DIGDI) ( Supplementary Fig. 6 ). Classifying the P. gaboni var genes with the VARdom server returned 8, 3, 1 and 1 hits to the DBLe, DBLz, DBLb and DBLg domains, respectively. As those results are different to the obtained alignment, we assume that the domains are too divergent to be classified with the VARdom server. Polymorphism versus divergence tests Amino acid repeats and low complexity regions in genes were identified by blasting each protein against itself. Any amino acid repeats with an identity of at least 95% and longer than 20 amino acids were masked for subsequent analysis. To mask low complexity regions, we used the SEG programme (from NCBI BLAST). A multiple amino acid alignment was generated with MUSCLE [55] for each orthologous group (defined through the RATT transfer) of P. reichenowi and the five P. falciparum lab clones: 3D7, HB3, DD2, IT and 7G8. From the amino acid alignment, we generated a nucleotide alignment. We excluded orthologous clusters if one gene was a pseudogene (contains an internal stop codon or frameshift). Alignment positions with gaps were excluded, as well as masked regions. From the resulting alignments, we calculated HKA [16] , MK [18] and K a/ K s [56] values ( Supplementary Data 4 ). HKA values ( Supplementary Data 4–6 ) were calculated by counting the proportion of pairwise differences in the intraspecific samples (laboratory clones) and the interspecific comparison, averaging across all pairwise intraspecific comparisons to get the overall nucleotide diversity π , and taking the average of the comparison of each of the P. falciparum sequences versus PrCDC to get the nucleotide divergence K . The HKAr is the π / K ratio. Intergenic regions were also analysed between orthologous genes that shared gene order. These regions were identified by the gene on their left hand side ( Supplementary Data 5 ). Smith–Waterman alignments were performed using SSEARCH [57] and indels or gap positions were deleted. For the MK test ( Supplementary Data 4 and 7 ), the number of fixed and polymorphic positions was generated using previously described software [58] that also provides a P value. The MK skew is the log 2 (( N poly / S poly )/( N fix / S fix )), where N and S are the number of non-synonymous and synonymous sites, respectively, and fix and poly refer to fixed differences and polymorphisms, respectively; Supplementary Data 7 ). To calculate the K a/ K s ratio ( Supplementary Data 4 and 8 ), we took the cleaned alignments of the MK test, extracting the sequences of Pf 3D7 and Pr CDC. A PERL script used the Bio::Align::DNAStatistics module to calculate the K a/ K s values [56] . Erythrocyte invasion genes Loci containing erythrocyte invasion genes were manually inspected using the Artemis Comparison Tool ( Fig. 4 ) [48] . By inspecting mapped 3 kb mate pairs, the orientation of the Rh2 locus in Pr CDC was confirmed; with the locus in its new orientation, 3-kb mate pairs mapped evenly across the locus boundaries, whereas no 3-kb mate could be mapped when the locus was flipped to match the orientation in Pf 3D7. Accession codes: P. reichenowi and P. gaboni sequence data have been deposited in the European Nucleotide Archive (ENA) under the accession codes ERP000299 and ERP000135 , respectively. Raw reads of P. falciparum IT, Dd2, HB3 and 7G8 have been deposited in the ENA under the accession codes ERS013737 , ERS005005 , ERS010000 and ERS006631 , respectively. The assembled contigs are available under the following accession codes: CBXM010000001 to CBXM010002055 (for P. reichenowi ) and CBUG010000001 to CBUG010025756 (for P. gaboni ). The assembled and annotated genome scaffolds of P. reichenowi have been deposited in EMBL under the accession codes HG810406 to HG810777 . How to cite this article: Otto, T. D. et al. Genome sequencing of chimpanzee malaria parasites reveals possible pathways of adaptation to human hosts. Nat. Commun. 5:4754 doi: 10.1038/ncomms5754 (2014).